TH2 cells and their cytokines regulate formation and function of lymphatic vessels Lymphatic vessels (LVs) are critical for immune surveillance and involved in the pathogenesis of diverse diseases. LV density is increased during inflammation; however, little is known about how the resolution of LVs is controlled in different inflammatory conditions. Here we show the negative effects of T helper type 2 (T H 2) cells and their cytokines on LV formation. IL-4 and IL-13 downregulate essential transcription factors of lymphatic endothelial cells (LECs) and inhibit tube formation. Co-culture of LECs with T H 2 cells also inhibits tube formation, but this effect is fully reversed by interleukin (IL)-4 and/or IL-13 neutralization. Furthermore, the in vivo blockade of IL-4 and/or IL-13 in an asthma model not only increases the density but also enhances the function of lung LVs. These results demonstrate an anti-lymphangiogenic function of T H 2 cells and their cytokines, suggesting a potential usefulness of IL-4 and/or IL-13 antagonist as therapeutic agents for allergic asthma through expanding LV mediated-enhanced antigen clearance from the inflammatory sites. The circulatory system consists of two components, blood vessels (BVs) and lymphatic vessels (LVs) [1] , both are essential for homeostasis in healthy organisms and are involved in the pathogenesis of diverse diseases [2] , [3] . In contrast to BVs, lymphatic capillaries are composed of monolayered lymphatic endothelial cells (LECs), which are not ensheathed by pericytes or smooth muscle cells and have a discontinuous basement membrane containing portals for cells such as dendritic cells allowing them to enter the LVs [4] , [5] . LVs comprise a unidirectional network that absorbs protein-rich fluid from peripheral tissues and drains it into the venous circulation through a conduit system of initial, collecting vessels, lymph nodes (LNs), lymphatic trunks and ducts [6] , [7] , [8] . In addition to fluid homeostasis, LVs are also important for immune surveillance and absorption of dietary fats [9] . Under physiological conditions, LVs are mostly quiescent; however, proliferation or remodelling of LVs is observed during various pathological conditions such as inflammation, wound healing and tumour metastasis [3] , [10] , [11] , [12] . Identification of an LEC-specific transcription factor, prospero homeobox protein-1 (Prox-1), as well as lymphatic markers like LV endothelial hyaluronan receptor-1 (LYVE-1) and podoplanin, has facilitated investigation of LV’s role in various diseases. In particular, Prox-1 plays an essential role in the proliferation, maintenance and survival of LECs [13] , [14] , [15] . Recently, we reported a transgenic mouse that expresses green fluorescence protein (GFP) under the control of the Prox-1 promoter ( Prox-1-GFP ), in which GFP is expressed only in the lymphatic, but not in, the blood vascular endothelial cells [16] . Because lymphatic capillaries have a discontinuous basement membrane and maintain in very close contact with their microenvironment [17] , any cellular and cytokine variations in the microenvironment can affect LV structure and function. LV remodelling during inflammation is a complex process largely influenced by growth factors and cytokines secreted by several cell types. For example, lymphangiogenesis is primarily mediated by an increased vascular endothelial growth factor (VEGF) gradient in the microenvironment [12] , [18] , [19] , [20] . In contrast to VEGF, interferon (IFN)-γ, a primary cytokine secreted by T helper type 1 (T H 1) cells, has been identified as a strong anti-lymphatic factor in the inflammatory microenvironment [21] . However, different inflammatory conditions can lead to various types of T H cell differentiation, resulting in the release of diverse cytokines [22] . T H 2 cells predominantly secrete interleukin (IL)-4 and IL-13, potent pro-inflammatory cytokines that play critical roles in allergic diseases such as asthma [23] , [24] . Two unique receptors utilize the IL-4 receptor α (IL-4Rα) chain: The type 1 receptor is composed of a heterodimer of the IL-4Rα and the common γ (γc) chain, whereas the type 2 receptor is a heterodimer of the IL-4 Rα and the IL-13 receptor α 1 (IL-13 Rα1) chain [25] . IL-4 binds to the type 1 receptor, and both IL-4 and IL-13 bind to the type 2 receptor. Binding of IL-4 and/or IL-13 activates the Janus kinase (JAK)-signal transducer and activator of transcription (STAT) pathways, specifically JAK1 and STAT6 (ref. 26 ). It has been reported that IL-4 can be pro-angiogenic at low concentrations and under hypoxic conditions, and can have potent anti-angiogenic activity at high concentrations through the inhibition of corneal neovascularization and microvascular endothelial migration [27] . To date, no studies have reported the effect of T H 2 cells and their cytokines on LVs. Considering the effects of T H 2 cytokines on BVs, we hypothesized that IL-4 and/or IL-13 could also regulate the formation and/or function of LVs. The heterogeneous effects of inflammatory conditions and T cell-secreted cytokines on LV remodelling and function led us to question the effects of T H cell-associated cytokines on LV remodelling. In this study, we investigate the effects of T H 2 cells and their cytokines on LECs in vitro and on remodelling of LVs in mouse models of allergic asthma in vivo . Our results show that IL-4 and IL-13 have strong anti-lymphangiogenic effects not only affecting the density, but also the function of LVs. Furthermore, the anti-lymphangiogenic effects of IL-4 and IL-13 are predominant even in a pro-lymphangiogenic factor-rich environment, thus, the density of airway LVs is not increased in murine allergic asthma models. The finding that blockade of T H 2 cytokines can improve lymphatic function is important and clinically relevant as it suggests that enhanced lymphatics mediated-rapid clearance of antigens from inflammatory sites could be a means of preventing or treating allergic diseases. Negative regulation of Prox-1 and LYVE-1 by IL-4 and IL-13 Previously, we have demonstrated that IFN-γ, a major T H 1 cell-associated cytokine, is anti-lymphangiogenic [21] . To identify other anti-lymphangiogenic factors under different inflammatory conditions, we examined the effects of T H 2 cells and their cytokines. GFP + mouse LECs (mLECs) were purified from LNs of Prox-1-GFP transgenic mice [16] and their properties as LECs were confirmed ( Supplementary Fig. 1 ). To investigate the effect of T H 2 cytokines on LECs, we first examined whether receptors for T H 2 cytokines are expressed on mLECs and found that mLECs express γ c as well as IL-4 Rα and IL-13 Rα1 chains ( Fig. 1a ). Next we assessed the effect of IL-4 and IL-13 treatment on the mRNA expression of the LV markers Prox-1 and LYVE-1 in LECs. We found that recombinant IL-4 or rIL-13 treatment reduced the expression of Prox-1 and LYVE-1 mRNA by mLECs in a dose-dependent manner ( Fig. 1b,c ). Similar effects were also observed in human LECS (hLECs) treated with rIL-4 or rIL-13 ( Supplementary Fig. 2 ) as well as rIFN-γ treatment as shown previously [21] . Furthermore, the expression of Prox-1 protein was also diminished in response to IL-4 and/or IL-13 treatment ( Fig. 1d and Supplementary Fig. 3 ). We also investigated the putative signalling pathways that might be involved in the IL-4 and IL-13-mediated inhibition of Prox-1 expression. As previous studies have shown that JAK1 signalling occurs downstream of both IL-4 and IL-13 (ref. 26 ), we found that pretreatment with the JAK1 inhibitor [28] , piceatannol, partially restored Prox-1 expression in a dose-dependent manner ( Fig. 2 ). Taken together, these results indicate that IL-4 and IL-13 downregulate essential regulators of LECs through JAK1-mediated signalling. 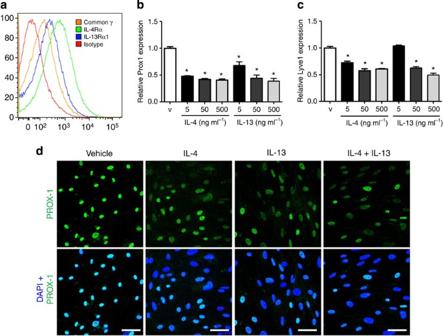Figure 1: Prox-1 and LYVE-1 expression following the treatment with IL-4 and IL-13. (a) IL-4 and IL-13 receptor expression on purified mLECs assessed by flow cytometry. Prox-1 (b) and LYVE-1 (c) mRNA expression levels following the treatment with indicated cytokines compared with vehicle (V)-treated mLECs were measured by real-time PCR. (d) Prox-1 expression following the treatment of cells with indicated cytokines (500 ng ml−1) was detected by confocal microscopy (blue: DAPI, green: Prox-1, scale bar, 50 μm). Data are presented as mean±s.e.m. and representative of three independent experiments (n=3), *P<0.05 compared with vehicle-treated group (non-parametric Mann–WhitneyU-test). Figure 1: Prox-1 and LYVE-1 expression following the treatment with IL-4 and IL-13. ( a ) IL-4 and IL-13 receptor expression on purified mLECs assessed by flow cytometry. Prox-1 ( b ) and LYVE-1 ( c ) mRNA expression levels following the treatment with indicated cytokines compared with vehicle (V)-treated mLECs were measured by real-time PCR. ( d ) Prox-1 expression following the treatment of cells with indicated cytokines (500 ng ml −1 ) was detected by confocal microscopy (blue: DAPI, green: Prox-1, scale bar, 50 μm). Data are presented as mean±s.e.m. and representative of three independent experiments ( n =3), * P <0.05 compared with vehicle-treated group (non-parametric Mann–Whitney U -test). 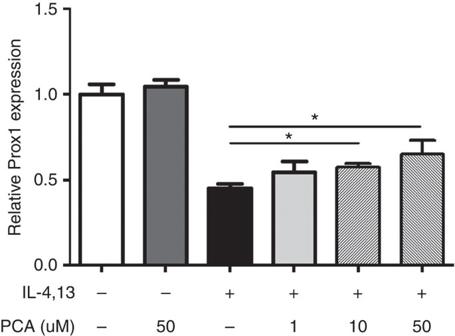Figure 2: Effects of JAK1 inhibitor on Prox-1 expression. Prox-1 expression in mLECs following the treatment with IL-4 and IL-13 along with the JAK1 inhibitor, piceatannol. Prox-1 expression levels compared with that of the vehicle-treated group was measured by real-time PCR. Data are presented as mean±s.e.m. and representative of three independent experiments (n=3), *P<0.05 compared with the indicated group (non-parametric Mann–WhitneyU-test). Full size image Figure 2: Effects of JAK1 inhibitor on Prox-1 expression. Prox-1 expression in mLECs following the treatment with IL-4 and IL-13 along with the JAK1 inhibitor, piceatannol. Prox-1 expression levels compared with that of the vehicle-treated group was measured by real-time PCR. Data are presented as mean±s.e.m. and representative of three independent experiments ( n =3), * P <0.05 compared with the indicated group (non-parametric Mann–Whitney U -test). Full size image Negative effects on lymphangiogenesis by T H 2 cytokines So far, our results have revealed that IL-4 and IL-13 downregulate LEC-specific transcription factor, Prox-1 and LEC marker, LYVE-1. Next we sought to investigate the functional consequences of the decreased expression of Prox-1 on LECs. To this end, we examined the effects of IL-4 and IL-13 on tube formation by LECs in vitro . While tube formation was easily observed as early as 6 h after LEC plating on Matrigel-coated wells under normal growth conditions, addition of rIL-4 and/or rIL-13 inhibited tube formation by mLECs for at least 24 h ( Fig. 3a,b ). Similarly, treatment with rIL-4 and/or rIL-13 also inhibited tube formation by hLECs in a similar way as rIFN-γ ( Fig. 3a,c and Supplementary Fig. 4 ). We also found that rIL-4 treatment inhibited tube formation by hLECs in a dose-dependent manner ( Supplementary Fig. 5 ). Together, these data suggest that IL-4 and IL-13 have an inhibitory effect on the adhesion and tube formation features of LECs. 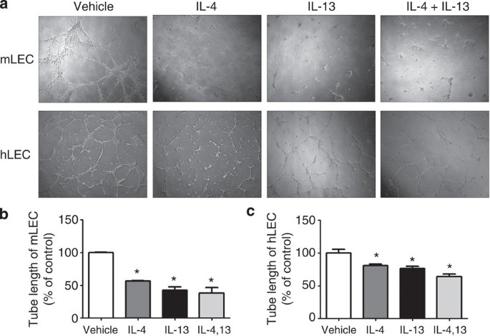Figure 3: Tube formation of LECs following the treatment with IL-4 and/or IL-13. Purified primary mLECs or hLECs (5 × 104cells) were cultured on Matrigel in EGM-2 media with indicated cytokines (500 ng ml−1) and 24 h later images were taken (a) and quantified (b,c). Data are presented as mean±s.e.m. and representative of three independent experiments (n=3), *P<0.05 versus the vehicle-treated group (non-parametric Mann–WhitneyU-test). Figure 3: Tube formation of LECs following the treatment with IL-4 and/or IL-13. Purified primary mLECs or hLECs (5 × 10 4 cells) were cultured on Matrigel in EGM-2 media with indicated cytokines (500 ng ml −1 ) and 24 h later images were taken ( a ) and quantified ( b , c ). Data are presented as mean±s.e.m. and representative of three independent experiments ( n =3), * P <0.05 versus the vehicle-treated group (non-parametric Mann–Whitney U -test). Full size image Both IL-4 and IL-13 are predominantly secreted by T H 2 cells and play a major role in the pathogenesis of allergic asthma [23] ; thus, we next tested the effects of T H 2 cells on tube formation by LECs. To examine whether cytokines secreted by T H 2 cells exert an inhibitory effect on mLECs, we first differentiated T H 2 cells from naïve CD4 DO11.10 T cells in vitro and co-cultured them with mLECs in a Transwell culture system. We confirmed polarized T H 2 cells produced large amounts of IL-4 and IL-13 without IFN-γ ( Supplementary Fig. 6 ). We found that tube formation by mLECs was significantly inhibited by T H 2 cell co-culture; these inhibitory effects were fully restored when neutralizing antibodies against IL-4 and IL-13 were added ( Fig. 4a,b ). Largely similar effects were observed with regard to the decreased Prox-1 expression in T H 2 cell co-cultured mLECs ( Supplementary Fig. 7 ). Taken together, these results indicate that the inhibitory effects of T H 2 cells on LECs were dependent on IL-4 and IL-13. 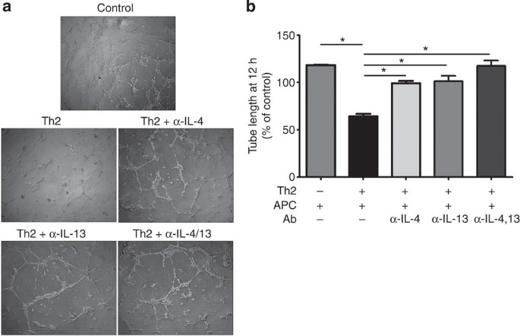Figure 4: Tube formation by mLECs co-cultured with TH2 cells. In a Transwell Matrigel assay,in vitropolarized TH2 cells (5 × 105cells) and/or APCs (5 × 105cells) were co-cultured with purified mLECs (5 × 104cells) with or without anti-IL-4 and/or anti-IL-13 antibodies. After 24 h, images were taken (a) and quantified (b). Data are presented as mean±s.e.m. and representative of three independent experiments (n=3), *P<0.05 compared with the indicated group (non-parametric Mann–WhitneyU-test). Figure 4: Tube formation by mLECs co-cultured with T H 2 cells. In a Transwell Matrigel assay, in vitro polarized T H 2 cells (5 × 10 5 cells) and/or APCs (5 × 10 5 cells) were co-cultured with purified mLECs (5 × 10 4 cells) with or without anti-IL-4 and/or anti-IL-13 antibodies. After 24 h, images were taken ( a ) and quantified ( b ). Data are presented as mean±s.e.m. and representative of three independent experiments ( n =3), * P <0.05 compared with the indicated group (non-parametric Mann–Whitney U -test). Full size image Increased lymphatic density by IL-4 and IL-13 neutralization On the basis on the inhibitory effects of T H 2 cells mediated by IL-4 and IL-13 on lymphangiogenesis in vitro , we expanded our investigation to determine the effect of these cytokines on LVs in vivo through a well-established allergen-induced asthma model [29] . Prox-1-GFP mice [16] were challenged with a mixture of Aspergillus protease and chicken egg ovalbumin (APO) allergen, symptoms of allergic asthma including airway hyper-responsiveness (AHR), airway inflammation and mucus hyper production were induced ( Fig. 5a–d and Supplementary Fig. 8 ). In addition, high levels of IL-4 and IL-13 secretion were detected in the bronchoalveolar lavage (BAL) fluid of allergen-challenged mice ( Fig. 5e,f ). Furthermore, when the recruited inflammatory cells in the lungs were re-stimulated with anti-CD3 and anti-CD28 antibodies, the production of IL-4 and IL-13 was significantly enhanced ( Supplementary Fig. 8 ). LVs proliferate during inflammation, thus we hypothesized that airway lymphatics would be increased in our experimental asthma model [3] , [30] . However, we could not detect an increase in the formation of lymphatics in the airways of APO allergen-induced asthmatic mice ( Fig. 6a,b ). Due to this unexpected observation, we hypothesized that inhibitory factors regulate lymphangiogenesis during allergic lung inflammation and focused on IL-4 and IL-13. In the allergen-induced asthma model, IL-4 and IL-13 were neutralized by the addition of neutralizing antibodies against these cytokines or IL-4Rα and the effects on LVs were examined. Blockade of both IL-4 and IL-13 or IL-4Rα increased the density of Prox-1 + LVs in the tracheas ( Fig. 6 ) and lungs ( Fig. 7 and Supplementary Fig. 9 ) of allergen-challenged asthmatic mice, and these inhibitory effects persisted for at least 6 days following the administration of the antibodies. Furthermore, to confirm that the anti-lymphangiogenic effect of IL-4 and IL-13 was responsible for the decrease in LV formation in allergen-induced asthmatic mice, APO allergen was administered to sublethally irradiated IL-4Rα-deficient mice reconstituted with wild-type (WT) bone marrow cells. Again, Prox-1 + LVs in the lungs of WT bone marrow-transplanted WT mice were unchanged while LVs in the lungs of WT bone marrow-transplanted IL-4Rα-deficient mice were increased following allergen challenge ( Fig. 8 ). Proliferation of LECs was inhibited with IL-4 and/or IL-13 treatment in vitro , and the diameter and numbers of sprouting LVs were also increased with blockade of both IL-4 and IL-13 in the tracheas of APO allergen-induced asthmatic mice ( Supplementary Fig. 10 ). Furthermore, considering cellular sources of IL-13, group 2 innate lymphoid cells (ILC2) could be another candidate; however, the numbers of ILC2 were not changed with or without blocking of cytokines nor compared with the saline group ( Supplementary Fig. 11 ). Thus, these findings confirm that the function of ILC2 is not related with at least in this model. Taken together, these results indicate that IL-4 and IL-13 inhibit lymphangiogenesis in vivo as seen in the airways of allergen-induced asthmatic mice by inhibiting the proliferation of LECs and enlargement of LVs. 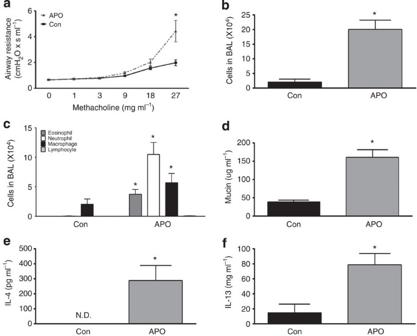Figure 5: Disease phenotypes of APO allergen-induced asthmatic mice. Airway hyper-responsiveness (AHR,a), inflammatory cells in BAL fluid (b), differential counting of inflammatory cells in BAL fluid (c), glycoprotein (mucin) quantification in BAL fluid (d), and the levels of IL-4 (e) and IL-13 (f) in BAL fluid were shown. Representative data are presented as mean±s.e.m. and representative of three independent experiments (n=5), *P<0.05 versus control (con) group (non-parametric Mann–WhitneyU-test). Figure 5: Disease phenotypes of APO allergen-induced asthmatic mice. Airway hyper-responsiveness (AHR, a ), inflammatory cells in BAL fluid ( b ), differential counting of inflammatory cells in BAL fluid ( c ), glycoprotein (mucin) quantification in BAL fluid ( d ), and the levels of IL-4 ( e ) and IL-13 ( f ) in BAL fluid were shown. Representative data are presented as mean±s.e.m. and representative of three independent experiments ( n =5), * P <0.05 versus control (con) group (non-parametric Mann–Whitney U -test). 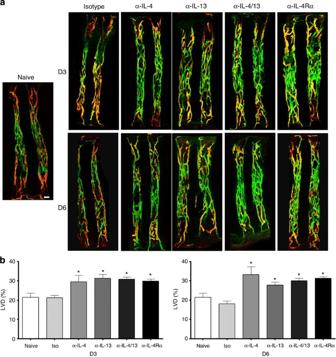Figure 6: Quantification of trachea LVs after allergen administration. Three or six days after final intranasal administration of allergen, LVs of tracheas were quantified in the group of mice receiving anti-IL-4 and/or anti-IL-13 or anti-IL-4Rα antibodies intratracheally. (a) Images were taken with a confocal microscope (red: LYVE-1, green: Prox-1, scale bar, 500 μm). (b) LV densities were quantified (D3: day 3, D6: day 6). Data are presented as mean±s.e.m. and representative of three independent experiments (n=4), *P<0.05 compared with the isotype antibody-treated group (non-parametric Mann–WhitneyU-test). Full size image Figure 6: Quantification of trachea LVs after allergen administration. Three or six days after final intranasal administration of allergen, LVs of tracheas were quantified in the group of mice receiving anti-IL-4 and/or anti-IL-13 or anti-IL-4Rα antibodies intratracheally. ( a ) Images were taken with a confocal microscope (red: LYVE-1, green: Prox-1, scale bar, 500 μm). ( b ) LV densities were quantified (D3: day 3, D6: day 6). Data are presented as mean±s.e.m. and representative of three independent experiments ( n =4), * P <0.05 compared with the isotype antibody-treated group (non-parametric Mann–Whitney U -test). 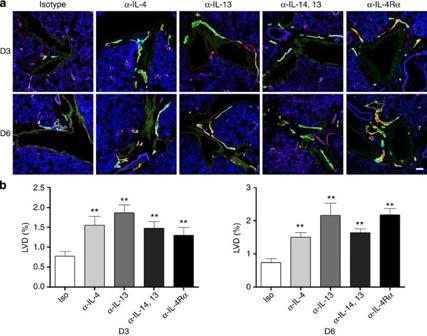Figure 7: Quantification of lung LVs after allergen challenge. Three (D3) or six (D6) days after the final intranasal administration of allergen, LVs of lungs were quantified following the intratracheal administration of anti-IL-4, anti-IL-13, anti-IL-4/IL-13 or anti-IL-4Rα antibodies. (a) Images were taken with confocal microscope (blue: PECAM-1, red: LYVE-1, green: Prox-1, scale bar, 100 μm). (b) LV densities were quantified. Data are presented as mean±s.e.m. and representative of three independent experiments (n=4), **P<0.005 compared with the isotype (iso) antibody-treated group (non-parametric Mann–WhitneyU-test). Full size image Figure 7: Quantification of lung LVs after allergen challenge. Three (D3) or six (D6) days after the final intranasal administration of allergen, LVs of lungs were quantified following the intratracheal administration of anti-IL-4, anti-IL-13, anti-IL-4/IL-13 or anti-IL-4Rα antibodies. ( a ) Images were taken with confocal microscope (blue: PECAM-1, red: LYVE-1, green: Prox-1, scale bar, 100 μm). ( b ) LV densities were quantified. Data are presented as mean±s.e.m. and representative of three independent experiments ( n =4), ** P <0.005 compared with the isotype (iso) antibody-treated group (non-parametric Mann–Whitney U -test). 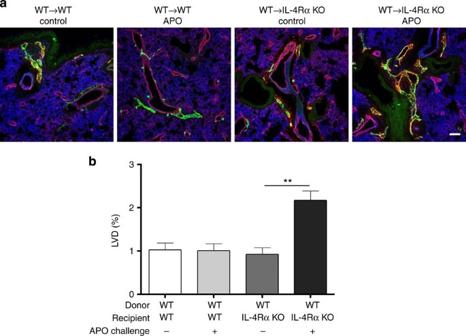Figure 8: Quantification of lung LVs after bone marrow transplantation. (a) Three days after the final intranasal administration of allergen, LVs of lungs were imaged by confocal microscopy (blue: PECAM-1, red: LYVE-1, green: Prox-1, scale bar, 100 μm). (b) LV densities were quantified. Data are presented as mean±s.e.m. and representative of two independent experiments (n=3), **P<0.005 compared with the indicated group (non-parametric Mann–WhitneyU-test). KO, knockout. Full size image Figure 8: Quantification of lung LVs after bone marrow transplantation. ( a ) Three days after the final intranasal administration of allergen, LVs of lungs were imaged by confocal microscopy (blue: PECAM-1, red: LYVE-1, green: Prox-1, scale bar, 100 μm). ( b ) LV densities were quantified. Data are presented as mean±s.e.m. and representative of two independent experiments ( n =3), ** P <0.005 compared with the indicated group (non-parametric Mann–Whitney U -test). KO, knockout. Full size image Enhanced lymphatic function by blockade of IL-4 and IL-13 Thus far, we have shown that T H 2 cells and their cytokines, IL-4 and IL-13, have an inhibitory effect on the formation of LVs and that this effect can be reversed with the neutralization of these cytokines. We next asked whether increased LV formation following T H 2 cytokine blockade correlates with the enhanced function of LVs. Thus, we first examined the trafficking of antigens from airways to draining LNs by administering red fluorescence protein (RFP)-labelled 2-μm polystyrene beads intratracheally followed by tissue imaging and bead quantification using confocal microscopy. The numbers of RFP-labelled beads in mediastinal LNs were increased in allergen-administered mice in which IL-4 and IL-13 were blocked as compared with the isotype antibody-treated control mice ( Fig. 9a,b ). Furthermore, to evaluate antigen clearance by LVs in airways, we administered high-molecular weight (two million daltons) fluorescein isothiocyanate (FITC)-conjugated dextran (FITC-dextran), which is widely used for examining the function of LVs, and calculated the recovery rate by quantifying fluorescence intensity [31] . Twenty-four hours post intratracheal administration of high-molecular FITC-dextran, allergen-challenged mice in which both IL-4 and IL-13 were neutralized showed significantly reduced amounts of FITC-dextran in BAL fluid compared with the control or isotype antibody-treated mice ( Fig. 9c ). Similar results were also observed using a direct fluorescence imaging system with In Vivo Imaging System (IVIS) and fluorescence-activated cell sorting (FACS) analysis ( Fig. 9d and Supplementary Fig. 12 ). Moreover, increased airway resistance of allergen-challenged mice was back to normal with blockade of both IL-4 and IL-13 ( Supplementary Fig. 13 ). Collectively, our results demonstrate that blockade of IL-4 and IL-13 increases not only the densities of LVs, but also their function. 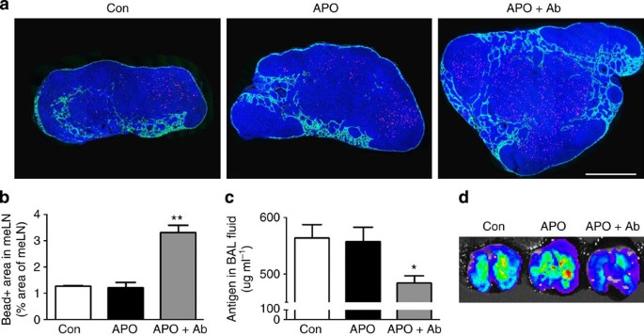Figure 9: Measurement of antigen delivery and clearance. (a) Beads in mLNs were imaged by confocal microscopy after the intratracheal administration of polystyrene beads (blue: DAPI, red: polystyrene beads, green: Prox-1). (b) Quantification of beads in mLNs. (c) After the lavage was performed, remaining FITC-dextran in the BAL fluid was quantified by luminometry. (d) FITC-dextran remaining in the whole lung was detected using the IVIS Lumina Imaging System. Con: control, which is the saline challenged group, APO: allergen-induced asthma treated with isotype antibodies, APO+Ab: allergen-induced asthma treated with anti-IL-4 and anti-IL-13 antibodies were shown in this figure (scale bar, 500 μm). Data are presented as mean±s.e.m. and representative of three independent experiments (n=4), **P<0.005 and *P<0.05 versus the isotype antibody-treated group (non-parametric Mann–WhitneyU-test). Figure 9: Measurement of antigen delivery and clearance. ( a ) Beads in mLNs were imaged by confocal microscopy after the intratracheal administration of polystyrene beads (blue: DAPI, red: polystyrene beads, green: Prox-1). ( b ) Quantification of beads in mLNs. ( c ) After the lavage was performed, remaining FITC-dextran in the BAL fluid was quantified by luminometry. ( d ) FITC-dextran remaining in the whole lung was detected using the IVIS Lumina Imaging System. Con: control, which is the saline challenged group, APO: allergen-induced asthma treated with isotype antibodies, APO+Ab: allergen-induced asthma treated with anti-IL-4 and anti-IL-13 antibodies were shown in this figure (scale bar, 500 μm). Data are presented as mean±s.e.m. and representative of three independent experiments ( n =4), ** P <0.005 and * P <0.05 versus the isotype antibody-treated group (non-parametric Mann–Whitney U -test). Full size image In this study, we investigated the roles of T H 2 cells and their cytokines, IL-4 and IL-13, in lymphangiogenesis using an in vitro LEC culture system and an allergic asthma model. We showed that T H 2 cells have anti-lymphangiogenic effects that are dependent on IL-4 and/or IL-13-mediated signalling. Furthermore, blockade of IL-4 and IL-13 increased LV density and function, as well as antigen clearance from the lungs and airways of allergen-induced asthmatic mice. LVs are the primary conduit for the migration of soluble antigens and antigen presenting cells (APCs) from the peripheral tissues to the LNs to initiate immune responses. LVs also facilitate the clearance of interstitial fluid and leucocytes from the sites where inflammation is being resolved [32] . In the present study, we showed that the function of LVs as a conduit for antigens and APCs was augmented following the neutralization of IL-4 and IL-13 in the airways of allergen-induced mice. The finding that lymphatic function could be improved by blockade of T H 2 cytokines is clinically relevant as it suggests that the rapid clearance of antigens from the inflammatory sites could be a means of preventing or treating allergic diseases. Previous strategies of treatment for experimental lymphedema induced by surgical damage have focused on pro-lymphangiogenic cytokines [33] , and in the clinic, treatments for lymphedema include lymphatic compression, exercise or surgical interventions [34] . Our data suggest that targeting anti-lymphangiogenic factors alone or in conjunction with other therapeutic approaches could be a new strategy for treating lymphedema. To date, there have been no reports in which the nature of LVs in the airways of asthmatics has been evaluated. Here we used Prox-1-GFP mice to monitor lung and airway lymphatics during allergic airway inflammation. It is well known that LYVE-1, a LV marker is not selective to LVs but also expressed by many kinds of myeloid cells and BVs in the lung [35] . Thus, the usage of Prox-1-GFP mice aids in the faithful visualization and quantification of LVs remodelling in airways and lungs. As asthma is an inflammatory disease, we reasoned that airway LVs would be increased in an allergen-induced asthma model; however, we failed to observe an increase in lymphatics in the airways of both APO allergen-induced asthmatic and OVA/alum-induced asthmatic mice ( Fig. 6 ). Thus, asthmatic airways were evaluated in mice in which WT bone marrow cells were transplanted into IL-4Rα-deficient mice where the density of LVs were not influenced by the factors other than IL-4 and IL-13. As expected, the density of LVs in the lungs of WT bone marrow-transplanted IL-4Rα-deficient mice was increased in response to allergen challenge. Furthermore, blocking IL-4 and/or IL-13 during allergic airway inflammation resulted in an enhanced density and function of airway lymphatics. Previously, McDonald’s group [36] showed that VEGF signalling axis is important in mouse models of chronic respiratory tract infection with Mycoplasma pulmonis . Although we did not evaluate indirect effects of VEGF signalling axis by blockade of IL-4 and L-13 in the allergic airway inflammation, direct effects of IL-4 and IL-13 on LECs in vitro strongly support direct inhibitory mechanisms of IL-4 and IL-13 on airway lymphangiogenesis. Surprisingly, lymphatics of tracheas, lungs and mediastinal LNs were all increased in the same manner following blockade of both IL-4 and IL-13 in allergic lung inflammation ( Figs 6 and 7 ). These results indicate that the anti-lymphangiogenic effects of IL-4 and IL-13 are predominant even in a pro-lymphangiogenic factor-rich environment. Recently, there have been reports that cytokines secreted by T cells affect LVs in various organs. One study showed that in a mouse-tail lymphedema model [37] , CD4 T cells negatively regulate lymphangiogenesis. Our group has also reported that IFN-γ secreted by T H 1 cells inhibits lymphangiogenesis in the draining LN in a lipopolysaccharide-induced skin inflammation model [21] . In contrast, IL-17 secreted by T H 17 cells promotes the growth of LVs in the corneas of mice with autoimmune dry eye disease [38] . In the present study, we demonstrated that IL-4 and IL-13 secreted by T H 2 cells inhibit lymphangiogenesis in a T H 2-dominant inflammatory condition. Extending our attention to human asthmatics, there is a report that lymphatics were decreased in the airway walls in cases of fatal asthma [39] . Conversely, in patients with allergic rhinitis, the densities of LVs were increased in allergic nasal mucosa compared with those in healthy nasal mucosa [40] . Notably, neither articles investigated the mechanisms underlying the observed phenomena. Here we report a negative regulation of lymphatics by T H 2 cells and dissect the underlying mechanism of this inhibition in an allergic lung inflammation model for the first time. In this study, we utilized an allergic asthma model in which the function of T H 2 cells and their cytokines plays a major role in the pathogenesis of the disease. However, clinical asthma and allergic rhinitis often show mixed forms of inflammation thus, T H 2 cytokine neutralizing agents have not been met with outstanding success in clinical trials until now. If we pursue chronic asthma where not only T H 2 cells but also other T H cells including T H 1 and T H 17 cells play an important role in the pathogenesis of the disease, then, we should consider the effects of those subsets of T H cells, too. Therefore, these issues should be investigated further to dissect pathogenesis of clinical asthma more precisely. Binding of IL-4 and/or IL-13 to their cognate receptors activates JAK–STAT pathways, especially JAK1 and STAT6 (ref. 26 ). In this study, we revealed that the JAK1 pathway is involved in IL-4 and IL-13-mediated Prox-1 downregulation. We also used the SABiosciences' proprietary database (DECODE, DECipherment Of DNA Elements) to search for binding sites of STAT6 in the promoter of the prox-1 gene and discovered that both human and mouse prox-1 genes contain a binding motif for STAT6 in their promoter regions. Furthermore, our group recently reported that STAT5 regulates Prox-1 expression by directly binding to the prox-1 promoter [41] . Thus, it is plausible that STAT6 could also be a transcriptional regulator of Prox-1. We also dissected the role of IL-4 and IL-13 in lymphangiogenesis, then linked these effects to the pathogenesis of asthma. Foreseeably, decreased antigen clearance caused by IL-4 and IL-13 could increase the time of antigen persistence, thereby prolonging inflammation in target organs such as lung. Notably, it should be pointed out that IL-4 and IL-13 themselves also play major roles in the pathogenesis of asthma. In our unpublished data, blocking IL-4 and IL-13 in an allergen-induced asthma model resulted in an amelioration of allergic asthma. To attribute this specifically to LVs, it is necessary to inhibit or to increase LVs selectively without altering levels of IL-4 and IL-13; a project that we are currently pursuing. In conclusion, our findings shed light on the previously unidentified roles of T cells as major regulators of LVs in the lungs and airways. In an inflammatory condition such as asthma, the levels of LVs were thought to be increased in the lungs similar to BVs; however, our findings show that LVs in the allergen-induced asthmatic lungs are not enhanced due to IL-4- and IL-13-mediated signalling in LECs. Considering the importance of LVs in many functional aspects of immunity, the anti-lymphangiogenic effects of these cytokines suggest that they play a pathogenic role in asthma. Mice The Prox-1-GFP BAC transgenic mice were described previously [16] . T-cell receptor transgenic DO11.10, IL-4Rα-deficient and WT mice were purchased from Jackson Laboratory (Bar Harbor, ME) and bred in our pathogen-free animal facility. Six- to eight-week-old female mice were used for this study. Animal care and experimental procedures were performed with the approval of the Animal Care Committee of KAIST. Histological, cytological and morphometric analyses These analyses were done as previously described [21] . Lungs were fixed in 4% paraformaldehyde, incubated in 20% sucrose solution, and embedded in a tissue freezing medium. Tracheas were fixed in 1% paraformaldehyde, washed, permeabilized with PBST (0.3% Triton-X 100 in PBS) and flat mount stained. Cultured LECs were fixed in 4% paraformaldehyde and permeabilized with PBST. After blocking with 5% donkey serum (Jackson ImmunoResearch, Grove, PA), the fixed tissues or LECs were incubated with the following primary antibodies: anti-mouse LYVE-1 (1 μg ml −1 , Angiobio Co., Del Mar, CA); anti-human Prox-1 (2 μg ml −1 , RELIATech, Braunschweig, Germany); anti-mouse CD31 (1 μg ml −1 , clone: 390, BioLegend, San Diego, CA); anti-mouse CD3 (1 μg ml −1 , 145-2C11, BD Biosciences, San Diego, CA) and anti-mouse B220 (1 μg ml −1 , RA3-6B2, BD Biosciences). After wash with PBS with Tween-20, sections were incubated with secondary antibodies (0.1 μg ml −1 ): FITC-conjugated anti-rabbit or anti-hamster; Cy3-conjugated anti-hamster, anti-rat or anti-rabbit; Cy5-conjugated anti-rabbit (all from Jackson ImmunoResearch). DAPI (1 μg ml −1 , Sigma-Aldrich, St Louis, MO) was used for nuclear staining. The samples were washed with PBS and mounted with fluorescence mounting medium (DAKO, Carpintería, CA). Fluorescence signals were visualized and digital images obtained using a Zeiss ApoTome inverted microscope or LSM 510 confocal microscope equipped with argon and helium-neon lasers (Carl Zeiss, Oberkochen, Germany). Prox-1 + LV density was measured at a screen magnification of × 100 by calculating the total sectioned area density of Prox-1 + vessel structures on digital fluorescence images using empirically determined threshold values, assessed in 4–5 mice per group. Values were obtained per millimeter square and expressed as relative densities. Purification of LECs from mouse LNs LNs from prox-1-GFP mice were digested in 2 ml of enzyme mix containing 0.2 mg ml −1 type-II collagenase (Worthington, Lakewood, NJ), 0.1 mg ml −1 DNase I (Worthington), and 0.8 mg ml −1 dispase (Invitrogen, Grand Island, NY) at 37 °C for 1 h with gentle agitation and pipetting 1–2 times to disrupt cell clumps. After digestion, cells were filtered through a 40-μm nylon cell strainer and cultured. After 5 days of culturing from digested LNs, cells were stained with phycoerythrin (PE)-conjugated anti-mouse CD45 antibody (0.5 μg ml −1 , clone: 30-F11, eBiosciences, San Diego, CA), allophycocyanin (APC)-conjugated anti-mouse CD31 antibody (0.5 μg ml −1 , 390, BioLegend) and CD45 − GFP + CD31 + LECs were sorted by flow cytometry (FACS Aria II, BD Biosciences). To assess receptor expression, PE-conjugated anti-mouse IL-13 Rα1 (1 μg ml −1 , 13MOKA, eBioscience), PE-conjugated anti-mouse common γ chain (0.5 μg ml −1 , TUGm2, BD Biosciences) and PE-conjugated anti-mouse IL-4 Rα (1 μg ml −1 , mIL4R-M1, BD Biosciences) antibodies were used. Data were analysed using FlowJo software (Tree Star, San Carlos, CA). Human dermal LEC culture Human dermal LECs were purchased from Cambrex (Cat # CC-2810, Walkersville, MD) and grown on a 0.1% gelatin-coated plate in 2% fetal bovine serum-containing endothelial cell basal medium-2 supplemented with growth factors (Lonza, Verviers, Belgium) at 37 °C. 80–90% confluent LECs (passaged fewer than 7 times) were used for all experiments. For treatment of LECs, recombinant human IL-4 (BD biosciences), human rIL-13, mouse rIL-4 and mouse rIL-13 (eBioscience) were added to the media at the indicated time points. To block JAK1, LECs were pretreated with piceatannol (Tocris, Ellisville, MO) in 0.1% DMSO-containing media 1 h before the addition of each cytokine and thereafter were cultured for 3 days. T H 2 cell differentiation CD4 T cells (2 × 10 5 ) were purified using positive selection from splenocytes using magnetic cell sorting (Miltenyi Biotec, Bergisch-Gladbach, Germany) and were co-cultured with 2 × 10 5 irradiated (3,000 rads) APCs (CD4 T cell depleted splenocytes), 10 μM OVA 323–339 peptide (ISQAVHAAHAEINEAGR), 1 ng ml −1 rIL-2 (BD biosciences), 1 ng ml −1 rIL-4, 10 mg ml −1 anti-mouse IFN-γ antibody (AN18, BD Biosciences) and 10 mg ml −1 anti-IL-12 antibody (C15.6, eBioscience) in RPMI-1640 medium supplemented with penicillin G (50 U ml −1 ), 50 μg ml −1 streptomycin, 2 mM L -glutamine (Invitrogen) and 10% fetal bovine serum (WelGene, Seoul, Korea) in a round-bottom 96-well plates (BD Biosciences) at 37 °C in a humidified atmosphere containing 5% CO 2 . After 5 days of culture, cells were expanded with 5 ng ml −1 rIL-2 and 5 ng ml −1 rIL-6 in 48-well plates (BD Biosciences) for 3 days. T H 2 cells were confirmed by the examination of IL-4 and IL-13 secretion by enzyme-linked immunosorbent assay (ELISA). One day before the co-culture, cells were re-stimulated with irradiated APCs and 10 μM of OVA 323–339 peptide in round-bottom 96-well plates. LECs and T H 2 cell co-culture One million T H 2 cells and/or APCs were added onto polycarbonate membrane cell culture inserts (0.4 mm pore, SPL life sciences, Korea). For neutralization, 20 μg ml −1 of anti-mouse IL-4 (11B11, BD Biosciences), anti-mouse IL-13 (eBio13A, eBioscience), anti-mouse IL-4 Rα (mIL4R-M1, BD Biosciences) and rat IgG2a κ isotype antibodies (BD Biosciences) were added. LECs tube formation assay LEC tube formation assay was performed in Matrigel (BD Biosciences). LECs (5 × 10 4 ) were seeded on Matrigel and images of tube formation and sprouting were taken using a light microscope with Deltapix pro-imaging system. The total lengths of tube-like structures (exceeding 20 μm in diameter) were measured and quantified. Real-time PCR Total RNA was extracted using Ribospin (GeneAll, Seoul, Korea) and complementary DNA was synthesized using SuperScriptIII First-Strand Synthesis System (Invitrogen). Quantitative real-time PCR was performed with the indicated primers using KAPA SYBR FAST qPCR kit in an iCycler (Bio-Rad, Hercules, CA) equipped with iQ5 (Bio-Rad). Data were analysed with Bio-Rad iQ5 Optical System Software (Bio-Rad). Average threshold cycle (Ct) was determined from triplicate reactions and levels of gene expression relative to GAPDH (Glyceraldehyde 3-phosphate dehydrogenase) were calculated. The following primers were used: hLYVE-1 5′- GCAAGGACCAAGTTGAAACAGCCTTG -3′ (forward), 5′- CTGGAATGCACGAGTTAGTCCAAGTA -3′ (reverse), hProx-1 5′- GCTCCAATATGCTGAAGACC -3′ (forward), 5′- ATCGTTGATGGCTTGACGTG -3′ (reverse), hGAPDH 5′- GGTGGTCTCCTCTGACTTCAACA -3′ (forward), 5′- GTTGCTGTAGCCAAATTCGTTGT -3′ (reverse), mLYVE-1 5′- GCAAGGACCAAGTTGAAACAGCCTTG -3′ (forward), 5′- CTGGAATGCACGAGTTAGTCCAAGTA -3′ (reverse), mProx-1 5′- CAATCACTTGAAAAAGGCAAAAC -3′ (forward), 5′- AAATTGCTGAACCACTTGATGAG -3′ (reverse), and mGAPDH 5′- AGGTCGGTGTGAACGGATTTG -3′ (forward), 5′- TGTAGACCATGTAGTTGAGGTCA -3′ (reverse). Western blot analysis After treatment with the indicated cytokines for 3 days, hLECs were lysed in radioimmunoprecipitation assay buffer (50 mM Tris, pH 7.5, 150 mM NaCl, 1% NP-40 and 1 mM ethylenediaminetetraacetic acid) containing phosphatase inhibitor cocktail (04906845001, Roche, Basel, Switzerland) and protease inhibitor cocktail (11697498001, Roche), incubated on ice for 30 min and then collected by centrifugation at 13,000 r.p.m. for 10 min. The lysates were separated by 8% SDS–PAGE and transferred onto the nitrocellulose membranes. After blocking with 5% BSA for 1 h, the membranes were incubated with anti-human Prox-1 (1 μg ml −1 , Cat # 102-PA32AG, RELIATech) antibody overnight at 4 °C followed by incubation with Horseradish peroxidase -conjugated anti-rabbit secondary Ab (1:4,000 dilution, Cell signaling) for 1 h at room temperature. Signals were developed with West Save Up (AbFrontier, Seoul, Korea), detected using LAS-1000 (Fujifilm, Tokyo, Japan) and the intensities of the bands were quantified using Multi Gauge (Fujifilm). Induction of experimental asthma Asthma induction was performed as described before [42] . Aspergillus oryzae protease allergen was purchased (Sigma-Aldrich) and reconstituted to 1 mg ml −1 in sterile PBS. Chicken egg ovalbumin (OVA, Sigma-Aldrich) was reconstituted to 0.5 mg ml −1 in sterile PBS. A. oryzae protease and OVA (APO) allergens were mixed 1:9 (v/v) immediately before administration. Mice were received four intraperitoneal sensitizations and single intranasal challenges every 4 days (day 0, 4, 8, 12 and 16) with 50 μl of allergen. For the neutralization of IL-4, IL-13 or IL-4Rα, indicated antibodies were administrated intratracheally 1 day after the final intranasal challenge. For lymphatic clearance experiments, FITC-conjugated dextran (2 million daltons; Sigma-Aldrich) or RFP-conjugated 2-μm polystyrene beads (Duke Scientific, Palo Alto, CA) were administrated intratracheally. Analysis of asthma phenotypes For all saline and allergen-challenged mice, AHR, BAL cytology, BAL glycoprotein assay and lung histopathology were determined as previously described [43] . Fourteen hours after the final intranasal challenge, mice were anaesthetized with pentobarbital sodium (Hanlim Pharma Co., Seoul, Korea, 60 mg Kg −1 ) and intubated using a 20-gauge cannula. After intubation, mice were connected via the endotracheal cannula to a flexiVent system (SCIREQ Inc., Montreal, Canada). To assess the airway responsiveness, mice were administered incremental doses of methacholine (Sigma-Aldrich) to the airway by nebulizer (SCIREQ), and the lung resistances were measured. The lung resistances were allowed to return to the baseline level between each dose of methacholine. Measurement of secreted glycoprotein in BAL fluid Glycoprotein mucin standard (derived from porcine stomach, Sigma-Aldrich) dissolved in PBS was diluted serially twofold. BAL fluid samples were diluted in PBS serially twofold beginning at a 1:100 dilution and 40 μl from each sample was transferred to flat bottom ELISA plate (Greiner, Kremsmunster, Austria) and incubated at 37 °C for 2 h or at 4 °C overnight. After washing, plates were blocked by the addition of 200 μl of 0.2% I-block and incubated at 37 °C for 2 h. After washing, 40 μl of biotinylated jacalin (Vector Laboratories, Burlingame, CA) diluted in PBS/Tween with 0.1% BSA to 5 μg ml −1 was added and the plates were incubated at 4 °C overnight. After another wash, 40 μl of alkaline phosphatase-conjugated streptavidin (BD Biosciences) diluted in PBS/Tween/BSA (1:1,000 dilution) was added and the plates were incubated at room temperature for 30 min. After a final wash, 70 μl of alkaline phosphatase substrate (5 mmol l −1 of p -nitrophenyl phosphate substrate in 0.1 mol l −1 alkaline buffer, Sigma-Aldrich) was added and developed until the standard curve was readily determined. The reaction was terminated by the addition of 40 μl of 0.5 N sodium hydroxide, and the optical density was measured at 405 nm by an ELISA plate reader (Bio-Rad). Transplantation of bone marrow cells Eight-week-old IL-4Rα-deficient or WT mice were sublethally irradiated with a single dose of 8.5 Gy and injected intravenously with a total of 1 × 10 7 bone marrow cells. Experiments were performed a minimum of 6 weeks after bone marrow transplantation. Quantification of fluorescence-conjugated polystyrene beads After allergic asthma induction, anti-IL-4 and IL-13 antibodies (25 μg) were administrated intratracheally 1 day after the final intranasal challenge. For lymphatic clearance assay, RFP-conjugated 1-μm polystyrene beads (Life technologies, Carlsbad, CA) were administrated intratracheally 3 days after antibody treatment. One day after beads treatment, single-cell suspensions from the lungs and mediastinal LNs of allergen-challenged mice were incubated with FITC-conjugated anti-CD11b (1 μg ml −1 , M1/70); APC conjugated anti-CD11c (1 μg ml −1 , HL3; all from BD Biosciences). Data were collected using a LSR Fortessa flow cytometer (BD Biosciences) and analysed using FlowJo software (TreeStar, Ashland, OR). Cell proliferation assay After treatment with indicated cytokines, cell pellets were collected for LEC proliferation analysis (MTT assay; Roche Applied Bioscience, Indianapolis, IN) according to the manufacturer’s instruction. Flow cytometry for quantification of CD4 T cells and ILC2 Single-cell suspensions prepared from the lungs of APO allergen-challenged mice were incubated with the indicated fluorochrome-conjugated antibodies and isotype controls: FITC-conjugated anti-CD4 (GK1.5); Pacific Blue-conjugated anti-CD3 (500A2); APC-Cy7-conjugated anti-Sca-1 (D7); PE-Cy7-conjugated anti-CD127 (A7R34); FITC-cocktail of the lineage marker (all antibodies from BD Biosciences except anti-CD127 from eBioscience). All antibodies were used at a concentration of 1 μg ml −1 . Data were collected using a LSRII flow cytometer (BD Biosciences) and analysed using FlowJo software (TreeStar). Statistical analysis Data were presented as mean±s.e.m. Non-parametric Mann–Whitney U -test was used for statistical analysis and P values (<0.05) were considered significant using GraphPad Prism Software V. 5.0 for Windows (GraphPad Software, La Jolla, CA). How to cite this article: Shin, K. et al . T H 2 cells and their cytokines regulate formation and function of lymphatic vessels. Nat. Commun. 6:6196 doi: 10.1038/ncomms7196 (2015).